CO2hydrogenation to high-value products via heterogeneous catalysis Recently, carbon dioxide capture and conversion, along with hydrogen from renewable resources, provide an alternative approach to synthesis of useful fuels and chemicals. People are increasingly interested in developing innovative carbon dioxide hydrogenation catalysts, and the pace of progress in this area is accelerating. Accordingly, this perspective presents current state of the art and outlook in synthesis of light olefins, dimethyl ether, liquid fuels, and alcohols through two leading hydrogenation mechanisms: methanol reaction and Fischer-Tropsch based carbon dioxide hydrogenation. The future research directions for developing new heterogeneous catalysts with transformational technologies, including 3D printing and artificial intelligence, are provided. Capturing carbon dioxide (CO 2 ) has emerged as an important method of mitigating its impact on environment [1] , [2] , [3] , [4] , [5] . However, this introduces the challenge of utilizing a large volume of captured CO 2 , which previously has not had any industrially viable uses at such a large scale. Realizing that, historically, fossil resources were produced via natural carbon-hydrogenation during photosynthesis, synthetic CO 2 hydrogenation is likely the best way to regenerate combusted hydrocarbons. While CO 2 hydrogenation is challenging due to the thermal stability of CO 2 , making reaction conversions low, considerable progress has been made towards converting CO 2 to single carbon (C 1 ) products (e.g., formic acid, carbon monoxide (CO), methane, and methanol) through direct hydrogen reduction or hydrothermal-chemical reduction in water [6] , [7] , [8] , [9] , [10] , [11] . Thermocatalytic hydrogenation of CO 2 to methane can be achieved easily at atmospheric pressure and high gas hourly space velocity (GHSV), and has been shown to achieve CO 2 conversion and CH 4 selectivity close to theoretical equilibrium values [12] . Hydrogenation to CO can be performed via the reverse water gas shift (RWGS) reaction. CO 2 -to-methanol (CTM) (CH 3 OH and MeOH) has already been industrialized in Reykjavik, Iceland using heterogeneous catalysis and geothermal energy [13] . In addition, catalysis for CO 2 hydrogenation to C 1 products has been widely studied with considerable progress [14] . Recently, significant progress has been achieved in heterogeneous catalytic hydrogenation of CO 2 to various high-value and easily marketable fuels and chemicals containing two or more carbons (C 2+ species), including dimethyl ether (DME) [15] , olefins [16] , liquid fuels [17] , and higher alcohols [18] . Compared to C 1 products, C 2+ product synthesis is more challenging due to the extreme inertness of CO 2 and the high C–C coupling barrier, as well as many competing reactions leading to the formation of C 1 products. However, C 2+ hydrocarbons and oxygenates possess higher economic values and energy densities than C 1 compounds. Therefore, this perspective mainly focuses on heterogeneous catalysis for CO 2 hydrogenation to high-value C 2+ products. Many reviews of heterogeneous catalytic hydrogenation of CO 2 have been published, organized according to using several approaches, including thermal, electrochemical, and photochemical hydrogenation [19] ; homogeneous and heterogeneous catalysts [20] ; and by their respective product distributions or catalysts employed [14] , [21] , [22] , [23] , [24] . Some are limited to C 1 products (e.g., methane or methanol) [14] , [25] . However, perspectives on heterogeneous catalytic CO 2 hydrogenation to C 2+ products are needed to guide scientists working in this area. Thus, this work is designed to help fill this gap and is organized to emphasize reaction mechanisms for producing C 2+ materials. The hydrogenation of CO 2 to C 2+ products mainly occurs via a methanol-mediated route or a CO 2 modified Fischer–Tropsch mechanism [17] , [26] . There are a variety of questions that need to be answered for each of these reaction mechanisms: what kinds of catalysts are beneficial for each route? How do the catalysts regulate product selectivity? What can be done to further enhance catalytic performance? What is the central challenge with catalysts for CO 2 hydrogenation to C 2+ products? To answer these questions, the catalysts for CO 2 hydrogenation to C 2+ species will be discussed based on the methanol-mediated route and the CO 2 modified Fischer–Tropsch route. Some experimental guidelines are provided to improve CO 2 conversion and to reduce C 1 byproducts. In addition, an outlook of transformational technologies for developing new catalysts is given in this work. Artificial intelligence (AI) is expected to guide the design and discovery of catalysis [27] , [28] , while 3D printing technologies are anticipated to be used to manufacture them on a large scale [29] . Methanol reaction based CO 2 hydrogenation Methanol (CH 3 OH) reaction based CO 2 hydrogenation can be realized by coupling two sequential reactions over a bifunctional catalyst. First, CO 2 and H 2 are converted to CH 3 OH over a partially reduced oxide surface (e.g., Cu, In, and Zn) or noble metals via a CO or formate pathway. Then, methanol is dehydrated or coupled over zeolites or alumina. Accordingly, bifunctional or hybrid catalysts are composed of a CH 3 OH synthesis catalyst and a CH 3 OH dehydration/coupling catalyst, which can convert CO 2 into high-value C 2+ compounds, including DME, hydrocarbons like gasoline, and light olefins. An efficient catalyst for these high-value C 2+ products should be active for both CH 3 OH synthesis and dehydration/coupling under the same conditions (Fig. 1a , R1 – R4 ). CO_2 + 3H_2 →CH_3OH + H_2O
 (R1) 
    2CH_3OH→CH_3OCH_3 + H_2O
 (R2) 
    nCH_3OH + H_2 →CH_3( CH_2)_n - 2CH_3 + nH_2O
 (R3) 
    nCH_3OH→CH_2 = CH( CH_2)_n - 3CH_3 + nH_2O
 (R4) Fig. 1: CO 2 hydrogenation to fuels and chemicals via the methanol reaction mechanism. a Schematic for the reaction mechanism of direct CO 2 hydrogenation to C 2+ products over bifunctional catalysts. b Two possible reaction pathways for methanol synthesis. c Schematic for methanol conversion into hydrocarbons inside zeolites via the hydrocarbon-pool mechanism. Full size image In CO 2 hydrogenation to C 2+ compounds, the reactions of CO 2 to CH 3 OH and CH 3 OH to C 2+ compounds take place at 200–300 °C and 400 °C, respectively, over bifunctional catalysts. Therefore, investigation of the reaction conditions, catalyst properties, and catalytic performance for CO 2 to CH 3 OH and CH 3 OH to C 2+ products is necessary. Methanol As mentioned earlier, one of the possible targets of CO 2 hydrogenation is to convert CO 2 to CH 3 OH. Significant progress has been made in this area recently, especially in developing copper (Cu)- and indium (In)-based catalysts [30] , [31] . Recent publications have dealt with Cu–ZnO composites, whose CH 3 OH selectivity ranges from 30 to 70% at CO 2 conversions less than 30% under typical reaction conditions (temperature: 220–300 °C, pressure <5 MPa, H 2 /CO 2 = 3) [32] , [33] . By increasing the pressure to 36 MPa and H 2 /CO 2 molar ratio to 10, the single pass CO 2 conversion can be increased to 95.3% with 98.2% methanol selectivity over a Cu–ZnO–Al 2 O 3 catalyst [34] . When Cu nanoparticles (NPs) are encapsulated in metal organic frameworks (MOFs) and strongly interact with their secondary structural units, the resultant metal NPs@MOFs (e.g., Cu ⊂ UiO-66 [35] and CuZn@UiO-bpy [36] ) show enhanced activity and 100% CH 3 OH selectivity, while preventing the agglomeration of the Cu NPs. In addition, ZrO 2 is a noted promoter or support in Cu-based catalysts for CTM hydrogenation [37] , [38] . Indium-based materials have shown promise as alternatives for CO 2 conversion to methanol. Pure In 2 O 3 can convert 7.1% of CO 2 with 39.7% selectivity to CH 3 OH at 330 °C and 5 MPa [39] . A Pd/In 2 O 3 catalyst with many interfacial sites and oxygen vacancies enhances CO 2 adsorption, achieving CO 2 conversions of above 20% with a methanol space time yield (STY) of 0.89 g MeOH g cat −1 h −1 at 300 °C and 5 MPa [31] . In 2 O 3 /ZrO 2 catalysts significantly boost the methanol selectivity to 99.8%, with a CO 2 conversion of 5.2% and long-term stability of 1000 h under industrially relevant conditions [40] . Besides the Cu and In-based catalysts, great progress has also been achieved with ZnO–ZrO 2 solid solution catalysts, as well as Pd/Pt-based catalysts [41] , [42] , [43] . The ZnO–ZrO 2 solid solution catalysts have achieved CH 3 OH selectivities of 86–91% under a GHSV of 24,000 mL g −1 h −1 with high thermal stability after being tested for more than 500 h; it also shows a strong resistance to sulfur-containing molecules [31] . In 2014, Norskov’s group reported a Ni–Ga bimetallic catalyst for CO 2 hydrogenation to CH 3 OH at 0.1 MPa, whose STY reached 0.64 g MeOH g cat −1 h −1 at 210 °C [44] . Subsequently, a series of noble metal based catalysts, such as Ga–Pd [45] , Au–CeO X /TiO 2 [46] , and Pt–MoO X /Co-TiO 2 [47] , were developed to convert CO 2 to CH 3 OH at low pressure or low temperature. Similarly, Fan’s group achieved low-pressure CH 3 OH synthesis via another series of multiple-metal catalysts that included In 2 O 3 , like Ni–In–Al/SiO 2 and La–Ni–In–Al/SiO 2 , starting with a phyllosilicate precursor [3] , [48] , and achieving CH 3 OH STYs of above 0.011 g MeOH g cat −1 h −1 at 255 °C and 0.1 MPa. Dimethyl ether (DME) There has been rapid development in DME synthesis from CO 2 hydrogenation using CH 3 OH synthesis catalysts hybridized with CH 3 OH coupling catalysts [15] . The effect of promoters, supports, and synthesis conditions have been explored [42] , [43] , [49] . For example, the acidic sites on γ-alumina surfaces and the CuAl 2 O 4 spinel phase can be regulated by promoters like gallium or zinc oxides, resulting in higher stability for Cu NPs during CO 2 -to-DME [49] . To date, CO 2 conversion and DME selectivity mostly vary between 35–80% and 5–50%, respectively [15] , but CO 2 conversion can reach up to 97% at 280 °C over a Cu–Zn–Al/HZSM-5 catalyst by drastically increasing the reaction pressure (to 36 MPa) [34] . In addition, interesting results have been reported on core–shell structured hybrid catalysts with the MeOH synthesis catalysts at the core and the MeOH dehydration catalysts forming the shell [50] , [51] . Compared with traditional hybrid catalysts prepared by physically mixing the components, these novel core–shell catalysts have received much attention in the literature due to their unique structures and ability to valorize CO 2 by improving conversion and DME selectivity. Light olefins, aromatics, and gasoline MeOH can not only be dehydrated to DME, but also serve as an intermediate to synthesize hydrocarbon chains, (CH 2 ) n , and final products, such as olefins, aromatics, and gasoline. As mentioned above, defective indium oxide (In 2 O 3 ) with oxygen vacancies is shown to be effective for CO 2 hydrogenation to CH 3 OH, while In 2 O 3 mixed with SAPO-34 is attractive for efficient CO 2 conversion to CH 3 OH and subsequent selective C–C coupling of CH 3 OH to form light olefins [52] . The addition of Zr into In 2 O 3 is helpful for creating more oxygen vacancies, enhancing CO 2 chemisorption and stabilizing both surface intermediates and active In NPs [53] , [54] . Similarly, a high yield of light olefins can also be achieved by composite catalysts, such as ZnZrO [16] , ZnGaO [55] , and CuZnZr [56] mixed with SAPO-34. 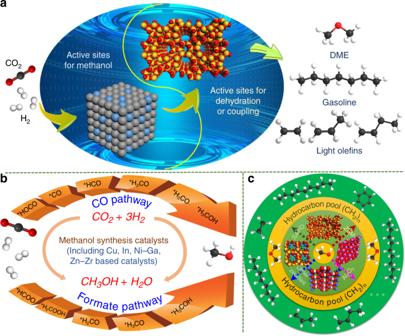Fig. 1: CO2hydrogenation to fuels and chemicals via the methanol reaction mechanism. aSchematic for the reaction mechanism of direct CO2hydrogenation to C2+products over bifunctional catalysts.bTwo possible reaction pathways for methanol synthesis.cSchematic for methanol conversion into hydrocarbons inside zeolites via the hydrocarbon-pool mechanism. As shown in Table 1 (Entries 1–5, 9–13), the selectivity of light olefins, represented by the C 2 –C 4 = column in the table, can be as high as 90%, while the CH 4 selectivity is less than 5% of the hydrocarbon products with 15–30% CO 2 conversions over most bifunctional catalysts tested, which deviates from the Anderson–Schulz–Flory (ASF) distribution. [52] , [54] This result is a significant breakthrough in the synthesis of light olefins. When the zeolite is changed from SAPO-34 to HZSM-5, more C 5+ compounds are produced than light olefins. A 78.6% selectivity of gasoline-range hydrocarbons, with only 1% CH 4 selectivity, was obtained from the tandem In 2 O 3 /HZSM-5 catalyst [26] . When In 2 O 3 is replaced by ZnAlO x or ZnZrO, CH 3 OH is synthesized on the metal oxide surface and then converted to olefins and aromatics inside the HZSM-5 pores with an aromatic selectivity of 73%, which is attributed to a shielding of the external Brønsted acid sites of HZSM-5 by ZnAlO x [57] . Therefore, the type of product is affected by both the character of the metal oxides and the geometries of the zeolites that determine the confinement of the hydrocarbons. Furthermore, as mentioned previously, catalysts with product yields exceeding the ASF distribution limit were recently reported that follow the methanol reaction mechanism-based CO/CO 2 hydrogenation. However, fundamental understanding of this ASF distribution deviation is still lacking. Jiao et al. [58] observed that ketene (CH 2 CO) can be formed from the reaction between surface CO and CH 2 species, blocking the surface polymerization, and thus breaking the ASF distribution. Another important reason suggested for the reported ASF distribution deviation is the use of bifunctional catalysts with two types of active sites. Table 1 Representative catalysts and their performance for hydrogenation of CO 2 to C 2+ species. Full size table Reaction mechanisms For most catalysts, the rate-determining step for methanol synthesis is CO 2 activation ( R1 ) [59] , [60] , which includes chemisorption of CO 2 and electron transfer from the catalyst to CO 2 [11] , [61] . Density functional theory (DFT) calculations have shown that different catalysts activate CO 2 through electron transfer between different orbitals [62] . For example, in PtCo-based catalysts, carbon in the CO 2 tends to bind to the Pt sites with an η 1 -C Pt bonding mode, while the O in the CO 2 prefer to combine with the reduced M δ+ cations in metal oxides with η 1 -OM δ+ configuration [63] . In addition, oxygen vacancies on metal oxide surfaces and Lewis acid sites have also been shown to enhance CO 2 activation [37] , [55] , stabilize intermediates [64] , and reduce sintering [52] . DFT calculations reveal that an oxygen-defective surface could be created through direct thermal desorption or exposure to a reducing agent [54] . After activation, CO 2 proceeds to form methanol, most likely via a formate intermediated pathway. The use of DFT and ab initio molecular dynamics sampling techniques on Cu–ZnO [32] , Cu–Pd [42] , [65] , In [66] , and Ga [48] , [67] catalysts suggest that methanol synthesis occurs via a formate intermediate (See Fig. 1b ). However, while calculations for Cu–ZnO interfacial sites suggest a formate intermediate [32] , calculations for the near surface regions suggest a CO intermediated pathway [68] . In addition, the calculations indicate that H 2 O produced in situ from both RWGS and CH 3 OH formation on Pd incorporated Cu catalysts accelerates CO 2 conversion to methanol by reducing the kinetic barriers by 0.2–0.7 eV for O–H bond formation steps [42] , [65] . On In-based catalysts, defective In 2 O 3 surfaces have different CO 2 activation barriers [66] . The synthesized methanol can then be transformed into high-value C 2+ compounds, including DME, lower hydrocarbons, and gasoline via the hydrocarbon-pool mechanism in which an organic center is trapped in the zeolite pores and acts as a co-catalyst, as depicted in Fig. 1c [26] , [69] , [70] . The DFT results indicate that the rate-determining step is generally CO 2 activation during conversion to methanol over the hybrid catalysts, whose ΔG 0 at 320 °C reaches 47 kJ/mol, which is much higher than that of the subsequent dehydration reaction (e.g., ΔG 0 = −87 kJ/mol for methanol to xylene at 320 °C) [71] , [72] ; thus, an efficient CH 3 OH synthesis catalyst is beneficial for the subsequent formation of C 2+ compounds. As indicated above, the bifunctional catalysts consist of CH 3 OH synthesis and dehydration catalysts. However, is the bifunctional catalyst mechanism also the simple sum of the two individual reactions? Li et al. [16] estimated the CH 3 OH selectivity based on the hydrocarbon selectivity for a hybrid catalyst and found that it was much higher than that for ZnZrO alone. This result clearly indicates that the products from the bifunctional catalysts are not a simple sum of the two individual reactions, and these two catalysts have a large synergistic effect. Thus, further study on the direct CO 2 hydrogenation to C 2+ products over bifunctional catalysts is still desirable. Fischer–Tropsch synthesis (FTS)-based CO 2 hydrogenation Heterogeneous FTS-based CO 2 hydrogenation can be realized in either one or two reactors, although the single reactor process dominates. The direct one-reactor conversion system has drawn much attention due to its ease of operation and thus lower CO 2 conversion cost. This process integrates the reduction of CO 2 to CO via the RWGS reaction and hydrogenation of CO to hydrocarbons via FTS. An efficient catalyst for generating C 2+ products, which generally refer to light olefins, liquid fuels, and higher alcohols, should be active for both RWGS and FTS under the same conditions (Fig. 2a , R5 – R7 ). The product distribution can be wide, depending on the structure and composition of the catalysts. Iron (Fe), cobalt (Co), and ruthenium (Ru) based supported catalysts, with appropriate promoters, are predominantly used in this area. nCO_2 + ( 3n + 1)H_2 →C_nH_2n + 2 + 2nH_2O  ( CO_2 Hydrogenation)
 (R5) 
    Δ _RH_573K = - 128 kJ/mol
 
    CO_2 + H_2 →CO + H_2O  ( RWGS)
 (R6) 
    Δ _RH_573K = 38 kJ/mol;
 
    nCO + ( 2n + 1)H_2 →C_nH_2n + 2 + nH_2O  ( FTS)
 (R7) 
    Δ _RH_573K = - 166 kJ/mol
 Fig. 2: CO 2 hydrogenation to C 2+ products via the FTS-based mechanism. a Scheme of CO 2 modified FTS-based catalytic mechanism. b – d CO 2 hydrogenation via the FTS mechanism for production of light olefins, liquid fuels, and higher alcohols [76] , [77] , [78] , [91] , [98] . e Synthesis strategy for an Fe-based catalyst. (Reprinted with permission from Ramirez et al. [83] . Copyright (2018) American Chemical Society). f Selective production of aromatics from the CO 2 hydrogenation process over a ZnFeO x – n Na/HZSM-5 catalyst. (Reprinted with permission from Cuiet al. [93] . Copyright (2019) American Chemical Society). Full size image (The values of Δ R H are reproduced from the literature [73] , [74] ). Prior to FTS, the RWGS reaction converts CO 2 to CO to form dissociatively adsorbed *CO precursor molecules on the catalyst surface. Therefore, an understanding of the reaction conditions and catalytic performance for the RWGS reaction is necessary. Since RWGS ( R6 ) is endothermic, it requires high temperatures for reasonable conversions. CO selectivity up to 100% can be achieved at 200–600 °C using the primary RWGS catalysts, such as Cu- and noble metal (Pt, Pd, Rh)-based catalysts, with CO 2 conversions up to 50% [75] . Light olefins Light olefins, including C 2 –C 4 alkenes, are important target products for the FTS-based CO 2 hydrogenation process. Fe-based catalyst systems are considered to be most suitable for olefin production by applying appropriate promoters, textural additives, or supports to form the required active sites for the different reaction stages. Fe and Co-based catalysts with alkali metal promoters (e.g., 35Fe–7Zr–1Ce–K [76] , Fe–Co/K–Al 2 O 3 [77] , and C–Fe–Zn/K [78] ) are reported to be highly active for FTS to produce C 2+ products [79] , [80] with as high as 57% selectivity at 40–60% CO 2 conversion (Fig. 2b ). The most effective promoters are alkali metals, especially Na and K, as they limit the formation of methane while improving the selectivity to C 2+ products [81] . Meiri et al. [82] pointed out that the introduction of potassium can stabilize the texture of the Fe–Al–O spinel, increase the surface content of Fe 5 C 2 , and strengthen CO 2 adsorption. In one study of fourteen different kinds of promoters added individually to MOF-derived Fe/C catalysts (Fig. 2e ), only K dramatically enhanced the olefin selectivity from 0.7 to 36% [83] . Martinelli et al. [84] concluded that the K-loading did not influence the CO 2 conversion, but increased the olefin/paraffin ratio and the average molecular weight of the products. Besides the alkali metals, other metals such as Cu, Zn, Ni, Zr, Mn, and Pt can also be used to modify Fe-based catalysts [83] . For example, bimetallic Fe–Cu/Al 2 O 3 catalysts can suppress CH 4 formation and thus exhibit higher amounts of C 2 –C 7 production compared with pure Fe/Al 2 O 3 catalysts [85] . Support material is another important factor that can influence catalyst activity and product selectivity by affecting the dispersion of active metals and the interactions between reactive intermediates and the support material. The support materials for Fe-based FT catalysts can be divided into metal oxides (e.g., ZrO 2 , CeO 2 , and Al 2 O 3 ) and carbonaceous materials (e.g., MOFs, mesoporous carbon, carbon nanotubes (CNTs), graphene, and organic precursors to mesoporous carbon). Wang et al. [86] studied several supports and found that a ZrO 2 supported (K-Fe/ZrO 2 ) catalyst exhibited the highest selectivity to lower olefins, while SiO 2 was not suitable for the CO 2 -FTS reaction. Since Fe carbides are generally considered to be the active phase in FTS catalysis, carbon materials are naturally considered as good support materials for Fe catalysts; indeed, they have demonstrated excellent catalytic performance for olefin synthesis. Carbon support materials can improve the dispersion of the active metals and lead to higher selectivity to olefins [87] . An Fe-based core–shell nanocatalyst with Fe 3 O 4 and Fe 5 C 2 in the core and partially graphitized carbon in the shell was prepared to efficiently convert CO 2 to C 2 –C 4 = olefins. The olefin/paraffin ratio was increased by carefully controlling the content of carbon to improve the accessibility of reactants to the active sites [88] . CNTs and graphene are also good carbon supports with superior thermal and chemical stability [87] , [89] . For example, a honeycomb-structured graphene (HSG) with a special meso-macroporous architecture was devised to confine K-promoted Fe NPs for the CO 2 -to olefins reaction. The FeK1.5/HSG catalyst can increase the selectivity of C 2 –C 4 = to 59.0% and the stability to 120 h, due to K promotion and HSG confinement effects [89] . Similarly, Ding et al. have successfully improved the catalytic activities by combining the K promoter and ZrO 2 support with sufficient oxygen defects [90] . C 5+ products Liquid fuels (e.g., gasoline and diesel) and other value-added chemicals (e.g., aromatics and isoparaffins) are also desired products from CO 2 hydrogenation via FTS. Jiang et al. [91] prepared Fe- and FeCo-based catalysts and achieved, when promoted with an appropriate amount of K, ≥54.6% CO 2 conversions and ≥47.0% C 5+ selectivity (Fig. 2c ). A Na–Fe 3 O 4 /HZSM-5 catalyst with three types of active sites was developed by Wei et al., demonstrating that 22% of CO 2 can be directly converted to gasoline with a selectivity of 78% [17] . When HZSM-5 was changed to HMCM-22, aromatization was suppressed, while isomerization was promoted due to the appropriate Brønsted acid properties of HMCM-22 and the special lamellar structure consisting of two independent pore systems. Thus, 57% selectivity of isoparaffins was obtained over the Na–Fe 3 O 4 /HMCM-22 catalyst, while the values over Na–Fe 3 O 4 /HZSM-5 and Na–Fe 3 O 4 were only 34 and 6%, respectively [92] . Similarly, aromatics are important feedstocks with applications in the synthesis of various polymers, petrochemicals, and medicines. ZnFeO x – n Na/HZSM-5 catalysts can achieve 75.6% selectivity to total aromatics at a CO 2 conversion of 41.2% (Fig. 2f ) [93] . Owing to superior ability for chain growth, stability, and lower activity for the WGS reaction, Co-based catalysts have also been applied to produce long-chain C 5+ hydrocarbons. Recently, a pure Co-based catalyst without promoters was reported to display high performance for both CO-FTS and CO 2 -FTS [94] , [95] . The Co/MIL-53(Al) catalyst was first found to exhibit 47.1% CO conversion and 68.6% selectivity to C 5+ products. When it was applied to CO 2 -FTS, 35.0% selectivity to C 5+ was still achieved at 260 °C. Furthermore, different kinds of promoters and support materials are employed to tune the product distribution towards heavier hydrocarbons. Shi et al. prepared a promoted Co–Cu bimetallic catalyst for CO 2 hydrogenation based on consideration of Cu as a popular RWGS catalyst. For example, with the introduction of Na as a promoter to a CoCu/TiO 2 catalyst, the CH 4 selectivity significantly decreased from 89.5 to 26.1%, while the C 5+ selectivity increased from 4.9 to 42.1%, with an excellent stability of more than 200 h [96] . He et al. [97] reported the bimetallic Co 6 /MnO x nanocatalyst with synergism between Co and Mn for 15.3% CO 2 conversion and 53.2% C 5+ selectivity. Higher alcohols Reports of higher alcohol (C 2+ OH) production are less prevalent compared to methanol and other C 2+ products of CO 2 hydrogenation. However, C 2+ OH alcohols have higher energy density and wider applications as fuel additives. The formation of higher alcohols is a parallel reaction competing with formation of hydrocarbons during the FTS process, resulting in much lower selectivity to C 2+ OH. Furthermore, the synthesis of C 2+ OH is difficult, as both C–C coupling and OH formation are required. Interestingly, water was found to enhance the selectivity of higher alcohols to 82.5% over a 1 wt% Pt/Co 3 O 4 catalyst (Table 1 , Entry 34) [98] . Moreover, the C 2+ OH selectivity was affected by the volume fraction of water, increasing dramatically with small amounts (<20 vol%) of added water, and then decreased slightly with further addition of water (Fig. 2d ). The promoting effect of water was attributed to assisting methanol dissociation to form more *CH 3 species. *CH 3 then can react with *CO to form *CH 3 CO, which will be further hydrogenated to ethanol (EtOH). Also, ordered Pd–Cu NPs, with charge transfer between Pd and Cu, are reported to efficiently convert CO 2 to ethanol with 92.0% selectivity (Table 1 , Entry 35). The rate-determining step of *CO hydrogenation to *HCO can be promoted on a Pd–Cu NPs/P25 catalyst, leading to lower *CO coverage and weaker *CO adsorption. Similarly, Cu–Fe and Zn–Fe interactions in the Fe-doped K/Cu–Zn catalyst have synergistic interactions, which can facilitate catalyst reduction and metal dispersion, as well as increase the yield of higher alcohols [99] . The reduction temperature can be regulated to obtain different phase compositions over the Co-based catalysts. For example, an alumina-supported catalyst reduced at 600 °C (CoAlO x −600) contained coexisting Co–CoO phases and exhibited 92.1% selectivity to ethanol at 140 °C, due to the formation of acetate intermediates from formate by insertion of *CH x [100] . Reaction mechanisms Although many successful catalysts have been developed for the CO 2 -FTS reaction, the nature of the active sites and reaction mechanism remain controversial. In view of the catalysts reported to date, the mechanism of the RWGS reaction can be assigned to either the decomposition of *HOCO intermediates or to direct C–O bond cleavage to produce *CO [75] . Ko et al. [101] pointed out that CO 2 can be activated to anionic CO 2 δ− through charge transfer from the pure and bimetallic alloy surfaces with bending of the structure and splitting of the π orbital. Both the adsorption energy of CO 2 δ− and the reaction energy for CO 2 dissociation are a linear function of adsorption energies of *CO and *O. To facilitate further *CO hydrogenation, the interaction between *CO and the catalyst interface need to be enhanced; otherwise, *CO is desorbed with concomitantly increased CO selectivity. According to the most-accepted reaction mechanism, during the FTS process, steps including *CO dissociative chemisorption on the active sites with hydrogen-assisted insertion to form *CH x intermediates, initiation of chain growth through the coupling of *CH x , and the termination of chain growth through further hydrogenation, dehydrogenation, or insertion of non-dissociatively adsorbed *CO happen successively on the catalyst surface (Fig. 2a ). *CO intermediates can be produced through the RWGS reaction, followed by the FTS reaction. According to modeling and kinetic analysis by Willauer et al., the RWGS reaction rate can reach 3.5 × 10 5 s −1 initially and decreases to 0.032 s −1 within 2 s, while the FTS reaction rate is zero initially and increases to 0.004 s −1 at 18.7 s [102] . The FTS reaction is the rate-limiting step due to the much lower reaction rate. The FTS reaction during the CO 2 hydrogenation process is limited by the reaction between the adsorbed CO and H 2 to form *HCO intermediates, as reported by Pour et al. [103] after evaluating different kinetic models and applying a genetic algorithm (GA) approach and the Levenberg–Marquardt (LM) method. Thus, efficient active sites for the FTS reaction are important for the whole CO 2 hydrogenation process. Also, chain propagation in FTS is still in dispute based on the basic C–C coupling mechanisms [104] . The most limiting process or factor during FTS-based CO 2 hydrogenation that should be addressed in future research may be affected significantly because of the various thermodynamic and physical properties of the reactions. For example, when using higher reaction temperatures (>300 °C), mass transfer appears to become the rate-limiting step instead of the surface reaction at relatively low temperatures [105] . Concerning the active sites in iron and cobalt catalysts, several phases are present and change dynamically during reaction. The catalyst transformation in structure and composition has several steps with their own kinetic regimes [106] . The reduced iron catalysts mainly consist of α-Fe and Fe 3 O 4 with extremely low activity at the beginning of FTS. Fe 3 O 4 is capable of activating CO 2 to CO via the RWGS reaction [81] , [107] . Then, the α-Fe reacts with the dissociatively adsorbed CO to form iron carbide (e.g., Fe 5 C 2 ), generating Fischer–Tropsch activity. Thus, the catalytic sites of iron carbides appear to be active for CO activation and chain growth [81] . Considering the different functions of iron species and the zeolites’ superior properties of acid sites for oligomerization/aromatization/isomerization, a multifunctional structure Na–Fe 3 O 4 /HZSM-5 catalyst was developed and achieved as high as 78% selectivity to gasoline, with only 4% methane generated [17] . Therefore, researchers need to focus not only on optimizing the composition and structure of the catalysts, but also on developing new catalytic systems with desired properties by using comprehensive approaches that can directly control the microstructures of the catalysts and be used for more accurately identifying the reaction pathways during FTS-based CO 2 hydrogenation. It is generally accepted that bulk Fe catalysts show insufficient catalytic performance and that the addition of promoters can enhance the selectivity to C 2+ products. However, the essential basis of the promotion effect remains unclear. More investigation needs to focus on the reaction mechanism. For example, the reaction pathways over Fe/Al 2 O 3 , Cu/Al 2 O 3 , and Fe–Cu/Al 2 O 3 catalysts are different, resulting in different product distributions [85] . Cu has high activity for the RWGS reaction instead of the CO 2 methanation reaction, leading to more surface *CO. Thus, bimetallic Fe–Cu/Al 2 O 3 catalysts form more CO, which leads to more C 2+ hydrocarbons compared to the Fe/Al 2 O 3 catalyst. Nie et al. also investigated the mechanism of CO 2 hydrogenation to methane and C 2 hydrocarbons over Fe(100) and Cu–Fe(100) surfaces and showed that the hydrogenation barrier of CH 2 * species is higher than those for C–C coupling and CH–CH* conversion to ethylene on Cu–Fe bimetallic catalysts (see Fig. 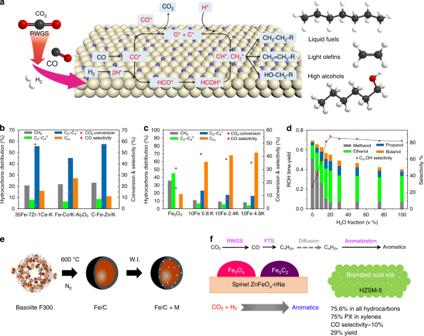Fig. 2: CO2hydrogenation to C2+products via the FTS-based mechanism. aScheme of CO2modified FTS-based catalytic mechanism.b–dCO2hydrogenation via the FTS mechanism for production of light olefins, liquid fuels, and higher alcohols76,77,78,91,98.eSynthesis strategy for an Fe-based catalyst. (Reprinted with permission from Ramirez et al.83. Copyright (2018) American Chemical Society).fSelective production of aromatics from the CO2hydrogenation process over a ZnFeOx–nNa/HZSM-5 catalyst. (Reprinted with permission from Cuiet al.93. Copyright (2019) American Chemical Society). 3 ) [108] , which results in a more selective process to ethylene. The addition of K to Fe–Cu/Al 2 O 3 catalysts can further inhibit methanation and enhance the production of olefin-rich C 2 –C 4 hydrocarbons by increasing the surface coverage of carbon [85] . DFT calculations show that the presence of K on Fe-based surfaces can enhance the CO 2 adsorption strength and reduce the CO 2 dissociation barrier (e.g., 2.36 eV for oct2-Fe 3 O 4 (111) versus 1.13 eV for K/oct2-Fe 3 O 4 (111)) [109] . Therefore, the introduction of promoters can modify the surface electronic features. Fig. 3: Mechanistic insight into C–C coupling over Fe-Cu bimetallic catalysts. a Mechanism of CO 2 hydrogenation to C 2 H 4 over a Cu–Fe(100) surface. b Reaction pathways for production of CH 4 , C 2 H 4 , and C 2 H 6 from CO 2 hydrogenation on Fe(100) and Cu–Fe(100) surfaces at 4/9 monolayer coverage. The kinetic barrier for each elementary step is given in eV. (Reprinted with permission from Nie et al. [108] . Copyright (2017) American Chemical Society). Full size image Methanol reaction based CO 2 hydrogenation The primary challenge in converting CO 2 to value-added products is low selectivity due to excessive formation of CO and the large amount of water (H 2 O) generated. CO and CH 4 are both formed due to partial reduction and cracking, respectively, during dehydration at the elevated temperatures (≥400 °C) generally employed for dehydration. To date, it has limited conversion (<30%) towards desired products (Table 1 , Entries 1–5, 7–13). In addition, H 2 O produced from CH 3 OH synthesis and dehydrative coupling further complicates separations and, in some cases, deactivates the catalyst. However, altering the zeolite structure has been shown to alter product distributions and increase selectivity to desired products, which was realized by increasing the space velocity during catalytic CO 2 hydrogenation over In 2 O 3 combined with zeolites [26] , [110] . Through the introduction of CO conversion promoters, such as In–FeK, In–CoNa, or CuZnFe/zeolites, bifunctional catalysts can be upgraded to reduce CO formation. In addition, these catalytic CO 2 conversion technologies face several other challenges, such as revealing the relationship between product type and molecular sieve type, increasing the CO 2 conversion and final product yield via improving the structures of bifunctional catalysts, as well as further elucidating the reaction mechanisms. More detailed information on these points is depicted below. First, more research on the zeolite properties is needed. By varying the zeolite structure, the product distribution can be better controlled. For example, HZSM-5 zeolite is selective towards DME and gasoline, whereas SAPO molecular sieves are preferred for light olefin generation. However, the structure-property relations between zeolite properties and CO 2 hydrogenation activity have not yet been systematically investigated. Because many variables and conditions exist during zeolites synthesis (e.g., synthesis template, crystallization temperature, and Si/Al ratio), the relationship between zeolite properties and CO 2 hydrogenation activity remains an active area of study [111] , [112] , [113] . Shape-selective catalysis was identified as a factor in these catalysts, as SAPO zeolite windows allowed only small linear hydrocarbons to pass, while H-ZSM zeolite windows allowed much larger branched and linear hydrocarbons to leave [114] . In addition, DFT calculations have linked density of surface Lewis acids and defects in the zeolite structure with dehydration activity [115] , [116] . Second, additional research on the structure of bifunctional catalysts is required. To improve CO 2 conversion and final product yield, the morphology and structure of the bifunctional catalysts should be optimized, rather than just making physical mixtures. The precise control of the desired morphology and structure of the catalyst is a significant and synthetically challenging task (see Fig. 4a–c ), as shown by the example of utilizing core–shell structures incorporating multiple-metal oxide cores to direct the growth of zeolite shells. Additionally, catalysts with core–sheath and lamellar structures are reported to exhibit high activity and stability for C=O bond hydrogenation [117] . Bifunctional catalysts can be assembled via layer-by-layer growth methods and probably exhibit better performance. Furthermore, efforts to improve important intrinsic factors, like the dispersion and crystallite size of active metals on methanol synthesis catalysts and the acid strength together with acid sites on the zeolites, as well as the methods of integration of the active components, should be made. As shown in Fig. 4d–f , different product distributions were obtained when the methanol synthesis catalyst and the zeolite were synthesized with different spatial arrangements [16] , [26] , [71] . The TEM and SEM images in Fig. 4g–i indicate that ZnZrO particles can be highly dispersed on the surface of HZSM-5 and maintain their own structures [16] , [26] , [71] . Sufficient physical mixing of the two components seems to be better than the granular form or a dual-bed separated in space by a layer of quartz sand. Fig. 4: The structure and performance of bifunctional catalysts. a – c Proposed structures of bifunctional catalysts. d – f Hydrogenation of CO 2 over bifunctional catalysts, which are integrated methanol synthesis catalyst and zeolites, with different spatial arrangements. (Adapted with permission from Li et al. [71] . Copyright (2019) Elsevier); Gao et al. [26] . 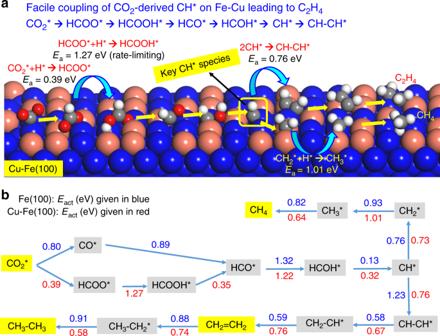Fig. 3: Mechanistic insight into C–C coupling over Fe-Cu bimetallic catalysts. aMechanism of CO2hydrogenation to C2H4over a Cu–Fe(100) surface.bReaction pathways for production of CH4, C2H4, and C2H6from CO2hydrogenation on Fe(100) and Cu–Fe(100) surfaces at 4/9 monolayer coverage. The kinetic barrier for each elementary step is given in eV. (Reprinted with permission from Nie et al.108. Copyright (2017) American Chemical Society). Copyright (2017) Springer Nature; Li et al. [16] . Copyright (2017) American Chemical Society). g – i TEM and SEM images of bifunctional catalysts. (Reprinted with permission from Li et al. [71] . Copyright (2019) Elsevier). Full size image Analyzing the integration between methanol synthesis catalysts and zeolites remains a challenge. DFT calculations may be the most efficient method to explore the interactions between CH 3 OH synthesis catalysts and dehydration catalysts. However, the information gained from DFT calculations can be limited because the systems studied are under idealized conditions, which are different from the ones in a packed bed reactor. As computing power with machine learning continues to increase, more complex and realistic catalytic systems can be modeled, which provides deep insight into the mechanism of CO 2 hydrogenation to olefins, such as the design of 3D nanocrystal tandem catalysts with multiple interfaces for CO 2 hydrogenation. FTS-based CO 2 hydrogenation The major obstacles of FTS-based CO 2 hydrogenation lie in the thermal stability of CO 2 and the complicated reaction mechanism with a wide product distribution. With the RWGS process being endothermic and FTS being exothermic, both need to be efficiently catalyzed under the same conditions, which sets a very strict requirement for the catalytic system. The designed catalysts should be effective for the RWGS reaction and also active enough for the subsequent FTS reaction. Different active sites must be precisely tuned and carefully dispersed on the support materials. These challenges will be discussed in view of different kinds of products: olefins, C 5+ hydrocarbons, and higher alcohols. The first, challenge to be discussed is production of light olefins. In spite of the promising results discussed, major challenges still remain. For example, the selectivity of C 2 –C 4 = can be above 80% for catalysts with methanol as the reactive intermediate, while only about 50% selectivity to C 2 –C 4 = is achieved on the catalysts for CO 2 conversion via FTS (Table 1 , Entries 14–21). The key to improve the C 2+ selectivity is to develop catalysts that have compatible bifunctional active sites for the two reaction steps, namely, *CO generation and subsequent *CO hydrogenation. The appropriately engineered reaction window is extremely important. The consequence of the incompatible activity of these two different types of active sites could be high CH 4 selectivity (~30%, Table 1 , Entries 14–21), as is suggested by the activation energy of RWGS being higher than that of CH 4 formation (81.0 and 59.3 kJ/mol, respectively) for Fe-based catalytic CO 2 hydrogenation [105] . As shown in Table 1 (Entries 1–8, 14–23), the reaction temperature (~320 °C) for the CO 2 -FTS process is lower than that for the methanol-mediated route (~380 °C). Thus, the CO selectivity (~30%) is dramatically reduced due to relatively low temperatures for the RWGS reaction, leading to improved hydrocarbon selectivity. Many researchers have tried to provide possible solutions for improving C 2+ selectivity by adjusting the structures and compositions of the catalysts. Specifically, development of enhanced promoters, supports, and experimental conditions have been attempted. For example, bulk Fe is favorable for methane formation; however, olefin and long-chain hydrocarbon production can be enhanced with the addition of promoters (i.e., alkaline promoters). Potassium, as an electronic promoter, can regulate the phase proportion of Fe 0 /FeO x /FeC x to maintain an optimum balance. The dissociative adsorption of *CO can be improved, while surface *H is decreased by donated electrons to the vacant d-orbital of Fe. The resulting higher C/H ratio favors chain growth and chain termination by forming unsaturated hydrocarbons [118] . Thus, a very important challenge is to increase the surface C/H ratio. Competitive adsorption between H 2 and CO occurs on the catalyst surface. The partial pressure of CO is always limited due the difficulty of converting CO 2 via the RWGS reaction. Since a high C/H ratio is desired to form unsaturated hydrocarbons, a possible strategy would be to enhance CO 2 activation and CO adsorption, while weakening H 2 adsorption [101] . In addition, the H 2 ratio in the feed gas should also be carefully chosen. To achieve good results from FTS-based CO 2 hydrogenation, more consideration is needed based on the characteristics of those reactions instead of imitation of the CO hydrogenation process. To increase selectivity to light olefins, further hydrogenation must be suppressed. Thus, synergy between the promoter and the support is suggested. For example, an Al 2 O 3 support can interact with a K promoter to form a KAlO 2 phase under calcination temperatures above 500 °C, which has been shown to suppress further hydrogenation of olefins [77] . To increase the synergistic effect, the active metal can be mixed with supports. A series of K-modified supports (activated carbon, TiO 2 , ZrO 2 , SBA-15, B-ZSM-5, and Al 2 O 3 ) were physically mixed with Fe 5 C 2 and tested for direct hydrogenation of CO 2 . The Fe 5 C 2 –10 K/α-Al 2 O 3 catalyst converted 40.9% of CO 2 with a selectivity of 73.5% to C 2+ products, containing 37.3% C 2 –C 4 = and 31.1% C 5+ [119] . A promising support for Fe-based catalysts is MOF-derived carbon materials. Some researchers have recently developed methods of using MOFs to fabricate carbon supported Fe-based catalysts [83] , [120] . Two Fe-MOF-derived catalysts have been reported for CO 2 hydrogenation, with high stability and selectivity to light olefins and liquid fuels [120] , [121] . However, the challenge of separating light olefins from unreacted CO 2 and H 2 remains. Increasingly advanced techniques and materials are required for their separation. The second, set of challenges are production of C 5+ products. These challenges are similar to those for the synthesis of light olefins, due to the shared fundamental reaction mechanism. The selectivity of C 5+ products is also comparable to that of light olefins synthesis (Table 1 , Entries 22–31). CO 2 hydrogenation to C 5+ products consist of multiple steps, including the RWGS reaction, C–C coupling, and acid-catalyzed reactions (oligomerization, isomerization, or aromatization). Therefore, cooperation between steps is required to develop an efficient and multifunctional catalyst. As zeolites are often used to incorporate the active sites, they generally undergo deactivation as a result of coke deposition. For example, the selectivity of isoparaffins over a Na–Fe 3 O 4 /HMCM-22 catalyst was reduced from ~60 to ~30% and the total acidity of HMCM-22 decreased from 0.200 to 0.032 mmol pyridine g cat −1 after 12 h of reaction time, which was attributed to coke formation and accumulation in the cavities and channels [92] . Thus, a big challenge for the synthesis of C 5+ products is to reduce coke deposition in the zeolites and to enhance the catalyst stability. As heavier hydrocarbons contain many components, it is difficult to precisely control a specific type of product. Zeolites with different framework topologies are suggested to regulate product distribution. In addition, in contrast to the CO-based FTS process, the reaction is fed with stable CO 2 molecules; therefore, the reformation of CO 2 from the produced CO via the WGS reaction is a thermodynamically favorable process, which limits CO 2 conversion [17] , [122] . One method to decrease the reformation of CO 2 from CO is to develop better multifunctional catalysts by employing appropriate promoters to facilitate the formation of iron carbide, which is known as the active catalyst for heavy hydrocarbon formation in FTS [96] , and to enhance the chemisorption and dissociation of CO 2 [123] . Also, by cycling reactants, CO 2 conversion is increased. Therefore, finding suitable multifunctional catalyst combinations or promoters and optimizing the reactors should be an attractive area of research in the future. Dual-promoter systems are usually designed to improve the RWGS reaction activity, while increasing FTS activity and C 5+ selectivity. Finally, there is a significant gap between the quality of synthesized liquid fuels and commercial gasoline. The octane number would be enhanced by developing catalysts that increase the fraction of isoparaffins in the gasoline. Finally, the challenges to produce higher alcohols are considered. For higher alcohols synthesis, the major obstacles are the formation and insertion of the hydroxyl group during the C–C coupling process in the presence of parallel reactions. This is made even more challenging since the formation pathways are different over Fe- and Co-based catalysts and the mechanisms are controversial. On K/Fe/N-functionalized CNT catalysts, alcohol synthesis was explained by the reaction between hydrocarbon species, such as alkylidenes (R-CH 2 -CH = ), and *OH, which forms from the dissociation of adsorbed CO (*CO) and H 2 (*H) [73] . *CO was hypothesized to react with *CH 3 species to form *CH 3 CO, which was then hydrogenated to form CH 3 CH 2 OH on a Na-Co/SiO 2 catalyst. To increase the yield of higher alcohols, efficient Co-based catalysts with more stable cobalt carbide (Co-Co 2 C) interfaces and/or Co-M alloy nanocrystals should be developed. Co 2 C is responsible for CO adsorption on the surface, whereas the Co metal is useful for CO dissociation and subsequent carbon-chain growth [124] . The synthesis of higher alcohols requires precise coordination between C–C coupling and OH formation, otherwise, more methanol or long-chain hydrocarbons would be produced. Also, the synergy of high metal dispersion and a high-density of hydroxyl groups on the supports can promote the selectivity to ethanol because the hydroxyls are able to stabilize formate species and protonate methanol [18] . The work from Fan’s group also indicates that metal oxyhydroxides, such as FeOOH [125] , TiO(OH) 2 [1] , and ZrO(OH) 2 [126] can accelerate the CO 2 sorption and desorption processes, thus reducing the energy required for CO 2 capture based on experimental and DFT calculations. These metal oxyhydroxides are likely catalyst candidates because they contain hydroxyl groups that should enhance CO 2 hydrogenation to higher alcohols. Transformational technologies for catalyst development Revolutionary material manufacturing, characterization, and evaluation technologies emerging in the new century may be instrumental for hydrogenating CO 2 to high-value products. However, these technologies are only beginning to be explored for their application to CO 2 hydrogenation. Thus, this perspective endeavors to fill in critical blanks. The keys are to discover alternative catalysts, modify current catalysts for CO 2 activation, develop methods to prepare specialized catalysts on a large-scale, and intelligently evaluate catalysts. Guided by reaction theories and the associated heterogeneous catalytic CO 2 hydrogenation experimental results, the feasibility of transformational technologies in three phases of CO 2 hydrogenation will be explored: catalyst preparation and modification, characterization, and AI-guided evaluation (see Fig. 5 ). Fig. 5: Scheme of AI-guided development of CO 2 hydrogenation catalysts. Phase I is to prepare and modify catalysts using 3D printing technologies and new material modification technologies, such as plasma, microwave, and ultrasound modification [135] , [137] , [138] . Phase II is to use advanced techniques to characterize the catalysts. Phase III is to perform AI-guided evaluation of the catalysts. Full size image Phase I is CO 2 hydrogenation catalyst preparation and modification. Conventional labor-intensive lab-based CO 2 hydrogenation catalyst preparation may be replaced by low-cost 3D-printing approaches to include characteristics of high mechanical strength and surface-to-volume ratio, with precise control of porosity, size, and shape [127] . The development of 3D-printed catalysts with designable and tunable structures is appealing and potentially useful for catalyst synthesis on a large scale. Although green 3D-printing has been utilized in preparing highly active, reusable, and stable catalysts for CO 2 removal, methane combustion, methanol to olefins conversion, syngas methanation, and N-aryl compound synthesis [128] , [129] , [130] , [131] , it has not been used for CO 2 hydrogenation or CO 2 conversion catalysts to date. Also, most of the printed catalysts are millimeter- to micrometer-sized materials, while nano- or atomic-sized catalysts are still challenging to print by existing 3D printing technology. As the functional components of active CO 2 hydrogenation catalysts are further studied (e.g., metals, promoters, and supports), more effort can be devoted to incorporating them into a fully integrated platform with diverse microstructures by 3D printing. As different spatial arrangements in bifunctional catalysts influence catalytic performance, 3D printing can assemble the components with multiple structures in their preferred configuration. Therefore, 3D printing provides an alternative approach for preparation of novel CO 2 hydrogenation catalysts, especially for synthesizing bifunctional catalysts. Realizing that AI has proven to be a great tool in a range of fields, including materials discovery and design [132] , the authors intend to apply a pioneering outlook with its application to CO 2 hydrogenation catalyst preparation, especially in combination with 3D printing technology. The 3D printing strategy already has advantages in potential scale-up manufacturing of catalysts, and AI technology would accelerate its application. AI-assisted 3D printing technologies can open new possibilities for the large-scale conversion of CO 2 . Also, new material modification technologies, such as microwave, ultrasound, and plasma treatments, have been suggested to modify catalysts for CO 2 activation, especially if the particle sizes or metal dispersion are affected by the 3D printing technologies. The utilization of unconventional modification tools in catalyst preparation and treatment can improve active phase dispersion to obtain a more uniform morphology with smaller particle sizes compared to the untreated catalysts [133] , [134] , [135] . Smaller particle size would enhance specific surface area and the exposed active sites available. The catalyst mechanical strength and the average basic site strength for CO 2 adsorption can be increased by microwave irradiation treatment, due to its better heat transfer [133] . Catalysts synthesized with the assistance of ultrasound, microwave, or plasma treatments have been employed in CO 2 hydrogenation and CO 2 /CH 4 reforming reactions [134] , [136] . These unconventional methods need high frequency and input power with reduced processing time [135] , [137] , [138] . In addition, the reactor can be constructed with plasma or microwave enhancement. The CO 2 -to-CH 3 OH reaction was accomplished in a plasma reactor without heating or adding pressure, generating a CH 3 OH selectivity of 53.7% and a CO 2 conversion of 21.2% over a Cu/γ-Al 2 O 3 catalyst [136] . Coupling of plasma and catalyst lowered the kinetic barrier and energy cost associated with conventional high temperature and high pressure processing. Therefore, the use of these new modification technologies before or after 3D printing can possibly remedy defects introduced by 3D printing technologies. Phase II is to characterize the CO 2 hydrogenation catalysts. New material characterization technologies, including in situ scanning transmission electron microscopy and temporal analysis of product reactors, coupled with qualitative and/or quantitative species identification, such as gas chromatography–mass spectrometry, are suggested for characterization of the catalysts prepared with state-of-the-art and transformational technologies. To date, in situ CO 2 -temperature programmed surface reaction and diffuse reflectance infrared Fourier transform spectroscopy have been applied widely to elucidate how CO 2 molecules dynamically interact with the catalyst. However, other characterization methods for heterogeneous catalysts under in situ conditions are challenging due to the lack of experimental facilities. Therefore, in the future, AI-assisted CO 2 hydrogenation catalyst characterizations are needed. Machine learning especially can bring advanced computational techniques to the forefront of characterization of heterogeneous catalysts. For example, machine learning can be used to help interpret experimental spectra. Although the imaging and spectroscopic results are complicated, it would be helpful to design new catalysts and link models and experiments by connecting these results to structure–function information [139] . Timoshenko et al. [140] have successfully deciphered the 3D geometric structure of supported Pt NPs with the use of X-ray absorption near-edge structure (XANES) spectroscopy and supervised machine learning. They solved the structures and reconstructed the morphology of Pt NPs just from the experimental XANES data using an artificial neural network. 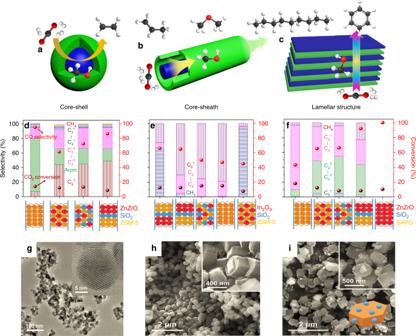Fig. 4: The structure and performance of bifunctional catalysts. a–cProposed structures of bifunctional catalysts.d–fHydrogenation of CO2over bifunctional catalysts, which are integrated methanol synthesis catalyst and zeolites, with different spatial arrangements. (Adapted with permission from Li et al.71. Copyright (2019) Elsevier); Gao et al.26. Copyright (2017) Springer Nature; Li et al.16. Copyright (2017) American Chemical Society).g–iTEM and SEM images of bifunctional catalysts. (Reprinted with permission from Li et al.71. Copyright (2019) Elsevier). 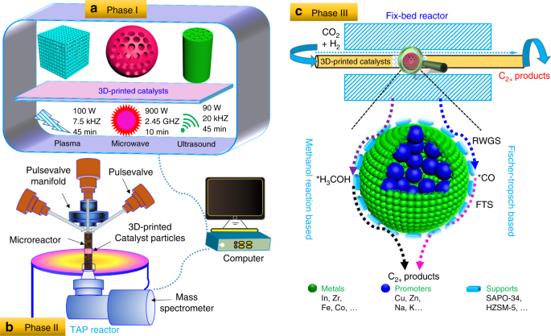Fig. 5: Scheme of AI-guided development of CO2hydrogenation catalysts. Phase I is to prepare and modify catalysts using 3D printing technologies and new material modification technologies, such as plasma, microwave, and ultrasound modification135,137,138. Phase II is to use advanced techniques to characterize the catalysts. Phase III is to perform AI-guided evaluation of the catalysts. Therefore, theoretical simulations can assist in obtaining more spectra and deconvoluting the structural characterization. Phase III is to perform AI-guided evaluation of CO 2 hydrogenation catalysts. The prospect of using AI for identification of reaction intermediates and pathways and establishing kinetic models would be promising. First, the AI-guided method is expected to predict catalytic performance and to discover promising catalyst candidates. AI-based catalyst evaluation might largely help predict and improve catalyst stability, which however will require more significant effort. Zahrt et al. [141] pointed out that machine learning has the potential to change the way chemists select and optimize catalysts. Some examples of recent results in AI-based catalyst evaluation follow. The hydrocarbon selectivities for DME conversion can be accurately predicted by an AI model with an R 2 greater than 0.98 compared to experimental results [142] . Several known and unknown electrocatalysts for CO 2 reduction and hydrogen evolution were identified from 1499 intermetallics by machine learning [27] . Specifically, 258 candidate surfaces among 102 alloys have been identified from 23,141 adsorption sites for the H 2 evolution reaction. Currently, it is inconvenient to characterize catalyst structures in situ during stability tests. Thus, in situ monitoring of the catalyst structure dynamics and transformation by AI would be beneficial. Second, we need more automatic, integrated, and flexible set-ups to evaluate catalysts. Third, data analysis could be performed and kinetic models evaluated with the help of AI. Numerous experimental data for CO 2 hydrogenation have been generated and this existing data should be reanalyzed. Kitchin suggests that machine learning can be applied to build models with more sophisticated methods [143] , generating new relevant data and calculated properties. Furthermore, it is crucial to identify reaction intermediates and pathways by AI. A simple syngas reaction on Rh(111) exhibits more than 2000 potential pathways [144] , in comparison with the more complicated CO 2 hydrogenation reaction routes that are strongly influenced by the various active centers. Hence, it is necessary to analyze the reaction mechanism by employing machine learning and DFT calculations. Finally, predicting relationships among the characteristics of the catalysts, such as Lewis acidity, CO 2 conversion efficiency, and product selectivity, with AI based on the available experimental data and DFT computation results will be helpful for discussing structure–function relationships and accelerating the discovery of catalytic mechanisms. Although AI offers many promising applications in CO 2 hydrogenation, robust and versatile AI is still in a primitive stage. A difficulty for AI development comes from the slowly developing applications of big data and a convenient language or software. Li et al. [28] pointed out that it is crucial and challenging to build additional criteria for screening and synthesizing catalysts, to quantify the uncertainties of machine-learning models, and to develop fingerprints of more sophisticated active sites with targeted functionalities. Also, more data for machine learning are required, including all reactions related to CO 2 , such as FTS, CO 2 /CH 4 reforming, and CO 2 hydrogenation. In conclusion, the collaborative efforts from experts and scientists in catalysis and materials design, machine-learning practitioners, and algorithm developers all over the world are needed to promote its development.